First enantioseparation and circular dichroism spectra of Au38clusters protected by achiral ligands Bestowing chirality to metals is central in fields such as heterogeneous catalysis and modern optics. Although the bulk phase of metals is symmetric, their surfaces can become chiral through adsorption of molecules. Interestingly, even achiral molecules can lead to locally chiral, though globally racemic, surfaces. A similar situation can be obtained for metal particles or clusters. Here we report the first separation of the enantiomers of a gold cluster protected by achiral thiolates, Au 38 (SCH 2 CH 2 Ph) 24 , achieved by chiral high-performance liquid chromatography. The chirality of the nanocluster arises from the chiral arrangement of the thiolates on its surface, forming 'staple motifs'. The enantiomers show mirror-image circular dichroism responses and large anisotropy factors of up to 4×10 −3 . Comparison with reported circular dichroism spectra of other Au 38 clusters reveals that the influence of the ligand on the chiroptical properties is minor. Chirality is ubiquitous in nature and has tremendous impact on biology, medicine, and pharmaceutical sciences. Whereas the origin of homochirality on earth is still unclear, it is now evident that many biological macromolecules are built from chiral building blocks. However, chiral assemblies can also emerge from achiral constituents. For example, achiral molecules may turn chiral on adsorption on a surface, even if the latter itself is not chiral [1] , [2] , [3] . In addition, achiral molecules can form chiral patterns on achiral surfaces [4] . This emergence of chirality is due to the restriction of the molecules to two-dimensional space on adsorption. This may lead to a reduced symmetry of the adsorbate complex or to chiral distortions of the molecule owing to its interaction with the surface. If chirality arises in such a way through the bonding of achiral constituents, a racemic mixture is obtained. Such phenomena have been studied on metal surfaces, where an adsorbate lattice can destroy the reflection symmetry of the metal surface underneath. Chiral domains are then formed on the surface with equal abundance of left- and right-handedness. This local chirality can be observed by scanning tunnelling microscopy [4] . An analogous situation was recently discovered on thiolate-protected gold particles or clusters. Jadzinsky et al . determined the structure of the gold nanocluster Au 102 ( p -MBA) 44 ( p -MBA: para -mercaptobenzoic acid) by X-ray crystallography [5] . An unusual bridged binding motif between gold and sulphur ('staple motif') was evidenced in which the sulphur atoms become chiral centres on adsorption. Moreover, it was found that the arrangement of the staples on the cluster surface forms a chiral pattern [5] . Because the p -MBA ligand used is achiral, both enantiomers are observed in the unit cell of the crystal. A similar situation is found for Au 38 (SR) 24 clusters (see below) [6] , [7] . The chirality of gold nanoparticles has recently become an intensively studied field of modern nanoscience as it opens new possibilities in catalysis and sensing applications [8] , [9] , [10] . The use of plasmon resonances in chiral metamaterials has been discussed and employed in several examples [11] , [12] , [13] , [14] , [15] . As gold nanoparticles exhibit localized surface plasmon resonances at diameters above ca 2 nm, their smaller analogues (up to ca 200 Au atoms) show interesting, molecular properties [16] . Among these small nanoparticles (in the following referred to as nanoclusters), thiolate-protected systems of the general formula [Au n (SR) m ] z (SR: thiolate; z: charge) have evolved as the most studied class, because of their extraordinary stability. Optical activity in Au:thiolate nanoclusters has first been observed by Schaaff and Whetten in 1998 (refs 17 , 18 ). Since then, numerous examples of more or less defined systems have been reported [19] . Protecting ligands include several derivatives of cysteine [10] , [20] , [21] , [22] , [23] as well as 'artificial' ligands such as binaphthyl systems [24] , [25] , [26] or other small organic thiolates [27] . Besides circular dichroism (CD) studies on the electronic transitions, the conformational analysis of the stabilizing ligand was demonstrated, using vibrational circular dichroism in the infrared [20] , [21] , [25] . Chiroptical properties in the ultraviolet-visible were found to be strongly size-dependent [24] . Also, it was shown that only a small fraction of enantiopure ligands in a mixed ligand system is sufficient to induce significant optical activity to the clusters [28] . Optical activity can result from a number of effects. Several models have been proposed to explain its origin in gold clusters, including the trivial case of using a chiral ligand (in this, the electrons in the gold core are trapped in dissymmetric electric fields) [29] ; a chiral footprint model (in analogy to classic surface chemistry, adsorption of a chiral ligand on the cluster surface perturbs the surface atoms in a chiral fashion) [20] , [30] and intrinsic core chirality [31] , [32] , as it was proposed that the equilibrium geometry of the core atoms is asymmetric. The importance of these different mechanisms for the optical activity observed in protected metal nanoclusters is difficult to assess, because, up to now, only for nanoclusters containing chiral enantiopure (or at least enantioenriched) ligands optical activity was reported. The above-mentioned staple motifs, which have been proposed earlier [33] , [34] , are an essential part of cluster structures. They can be thought as [thiolate-Au(I)] x -thiolate (x=1, 2) oligomers that bind in a bidentate fashion to the gold atoms of the cluster core. Staple-type binding was also identified for extended surfaces (self-assembled monolayers of benzenethiol and methylthiol on Au(111)) [35] , [36] . Such staples can be the source of chirality, as outlined above. The staple motif was also found in the crystal structure of [Au 25 (SCH 2 CH 2 Ph) 18 ] −1 and Au 38 (SCH 2 CH 2 Ph) 24 (refs 7 , 37 , 38 ). Similar to Au 102 , Au 38 shows intrinsic chirality by the arrangement of the staple motifs on the cluster surface. In contrast, this is not the case for Au 25 . A chiral arrangement of staples has also been proposed for Au 144 (SR) 60 clusters [39] . Au 38 (SCH 2 CH 2 Ph) 24 is of prolate shape, containing a face-fused biicosahedral Au 23 core and is protected by 3 short Au(SR) 2 and 6 long Au 2 (SR) 3 staples ( Fig. 1 ) [6] , [7] , [40] . The bare core can be idealized as of D 3h symmetry (in reality, slight distortions are found), which is lowered by the protecting staples to adopt a D 3 symmetry. The staples are arranged in a chiral fashion: the long staples are arranged in a staggered configuration of two triblade fans (composed of three staples), that either rotate clockwise or anti-clockwise (but both in the same sense, within one enantiomer), depending on the enantiomer. Moreover, the short staples at the equator of the cluster are slightly tilted with respect to the threefold axis, following the handedness of the long staples. 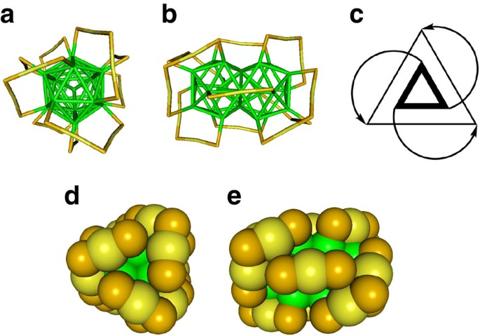Figure 1: Crystal structure of the left-handed enantiomer of Au38(SCH2CH2Ph)24. For clarity, the -CH2CH2Ph units were removed; yellow, gold adatoms; green, core atoms (Au); orange, sulphur. (a) Top view of the cluster; (b) side-view; (c) schematic representation highlighting the handedness of the cluster. The inner triangle represents the top three core atoms binding to the long staples. The arrows represent long staples and the outer triangle represent the core Au atoms binding to the 'end' of the staple. This representation is a top view along theC3axis, and the two triangles are not in one plane. (d) Top-view in space-filling representation mode; (e) side-view in space-filling representation mode. The structures were created using the crystallographic data provided in ref.7. Figure 1: Crystal structure of the left-handed enantiomer of Au 38 (SCH 2 CH 2 Ph) 24 . For clarity, the -CH 2 CH 2 Ph units were removed; yellow, gold adatoms; green, core atoms (Au); orange, sulphur. ( a ) Top view of the cluster; ( b ) side-view; ( c ) schematic representation highlighting the handedness of the cluster. The inner triangle represents the top three core atoms binding to the long staples. The arrows represent long staples and the outer triangle represent the core Au atoms binding to the 'end' of the staple. This representation is a top view along the C 3 axis, and the two triangles are not in one plane. ( d ) Top-view in space-filling representation mode; ( e ) side-view in space-filling representation mode. The structures were created using the crystallographic data provided in ref. 7 . Full size image In this contribution, we demonstrate for the first time that it is possible to separate the enantiomers of this Au 38 cluster covered with achiral thiolates (2-phenylethylthiolate) by a high-performance liquid chromatography (HPLC) column. A major prerequisite is the isolation of pure Au 38 cluster from the crude reaction product, as the employed thermal etching method usually yields polydisperse clusters [41] . This was achieved by gel permeation chromatography (GPC, or size exclusion chromatography, SEC). Successful enantioseparation enables us to measure optical activity for an enantiopure thiolate-protected gold cluster. The optical activity arising from the chiral arrangement of the staples is large. The anisotropy factors (ΔA/A) are the largest reported so far for thiolate-protected gold clusters, indicating the importance of the chiral pattern for the chiroptical response of such systems. Isolation and characterization of rac-Au 38 (SCH 2 CH 2 Ph) 24 Racemic Au 38 (SCH 2 CH 2 Ph) 24 was prepared and purified according to previously reported protocols [28] , [41] . Briefly, tetrachloroauric acid and L -glutathione were co-dissolved in water and methanol and reduced by sodium borohydride. The resulting precursor material was then dissolved in water and a mixture of acetone and 2-phenylethylthiol was added. A mixture of Au n (SCH 2 CH 2 Ph) m ( n =25–144, m =18–60), containing Au 38 (SCH 2 H 2 Ph) 24 , as major component was gained by heating the system to 80 °C. Excess thiol was removed by extensive methanol washing and the crude clusters were size-selected by gel permeation chromatography. The monodisperse racemic clusters were characterized by ultraviolet-visible spectroscopy and MALDI mass spectrometry ( Fig. 2 ) [42] , [43] ; the spectra are in agreement with previously reported data [41] . A single peak at 10,778 Da (calc: 10,778.08) and a characteristic fragmentation pattern in the mass spectrum indicates monodispersity based on the sensitivity of MALDI spectrometry. The unit cell of the crystal structure bears both enantiomers of Au 38 (SCH 2 CH 2 Ph) 24 , but the synthesis of the clusters involves the use of homochiral L -glutathione, and a chiral induction that might lead to an enantiomeric excess in Au 38 cannot be fully excluded. A CD spectrum was recorded showing no significant signals, suggesting that the Au 38 (SR) 24 nanoclusters used are a truly racemic mixture. 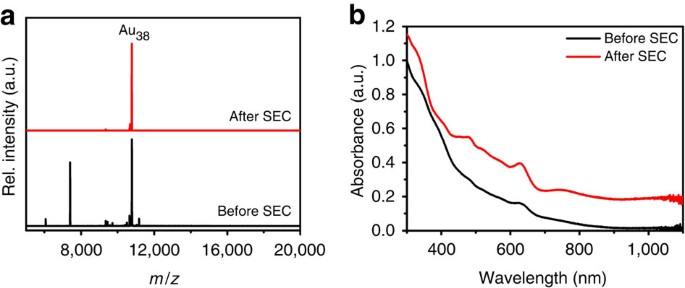Figure 2: Characterization ofrac-Au38(SCH2CH2Ph)24. (a) MALDI mass spectra of Au38(SCH2CH2Ph)24before (black) and after (red) size selection. The signals for Au40(SCH2CH2Ph)24(11,173 Da) and Au25(SCH2CH2Ph)18(7,391 Da) disappeared from the spectrum, indicating successful size exclusion. For a detailed description of this process, see ref.41. (b) Ultraviolet-visible spectra of Au38(SCH2CH2Ph)24before (black) and after (red) size selection. The absorption features of Au38are drastically enhanced. Figure 2: Characterization of rac -Au 38 (SCH 2 CH 2 Ph) 24 . ( a ) MALDI mass spectra of Au 38 (SCH 2 CH 2 Ph) 24 before (black) and after (red) size selection. The signals for Au 40 (SCH 2 CH 2 Ph) 24 (11,173 Da) and Au 25 (SCH 2 CH 2 Ph) 18 (7,391 Da) disappeared from the spectrum, indicating successful size exclusion. For a detailed description of this process, see ref. 41 . ( b ) Ultraviolet-visible spectra of Au 38 (SCH 2 CH 2 Ph) 24 before (black) and after (red) size selection. The absorption features of Au 38 are drastically enhanced. Full size image HPLC separation of rac -Au 38 (SCH 2 CH 2 Ph) 24 The racemic clusters were separated at room temperature using a chiral cellulose-based analytical HPLC column and hexane/isopropanol (80:20) as eluent. The eluting solutions were monitored by an ultraviolet detector at 380 nm. Two peaks well separated were observed at 8.45 and 17.45 min (enantiomers 1 and 2 according to increasing elution times, Fig. 3a ). The second peak is broadened and less intense compared with the first one, but integration gives identical peak areas to within the accuracy of the measurement. Runs at different temperatures (in the range of 10–25 °C) showed that separation is slightly better at lower temperatures. The ultraviolet-visible spectra of both peaks clearly show the distinct signature of Au 38 (SR) 24 clusters ( Fig. 3b ). 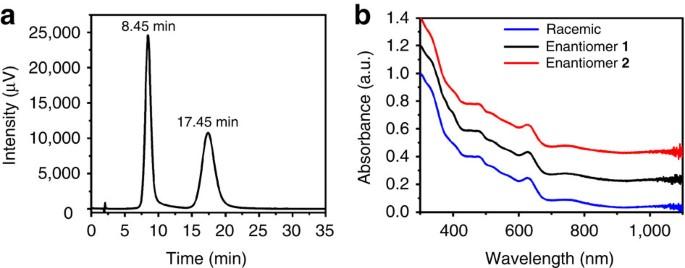Figure 3: HPLC-separation ofrac-Au38(SCH2CH2Ph)24. (a) HPLC-chromatogram of the enantioseparation ofrac-Au38(SCH2CH2Ph)24with the ultraviolet-visible detector at 380 nm. The peak at 8.45 min corresponds to enantiomer1; the second peak at 17.45 corresponds to enantiomer2. (b) Ultraviolet-visible spectra of enantiomers1(black) and2(red) and of the racemate (blue). The spectra were normalized at 300 nm and off-set for clarity. The well-known ultraviolet-visible signature of Au38is perfectly reproduced in all spectra, showing that the two collected fractions are composed of Au38(SCH2CH2Ph)24. Figure 3: HPLC-separation of rac -Au 38 (SCH 2 CH 2 Ph) 24 . ( a ) HPLC-chromatogram of the enantioseparation of rac -Au 38 (SCH 2 CH 2 Ph) 24 with the ultraviolet-visible detector at 380 nm. The peak at 8.45 min corresponds to enantiomer 1 ; the second peak at 17.45 corresponds to enantiomer 2 . ( b ) Ultraviolet-visible spectra of enantiomers 1 (black) and 2 (red) and of the racemate (blue). The spectra were normalized at 300 nm and off-set for clarity. The well-known ultraviolet-visible signature of Au 38 is perfectly reproduced in all spectra, showing that the two collected fractions are composed of Au 38 (SCH 2 CH 2 Ph) 24 . Full size image Circular dichroism of Au 38 (SCH 2 CH 2 Ph) 24 To confirm the separation of enantiomers, we collected the fractions according to the peaks over several HPLC runs and concentrated the combined solutions. CD spectra of these concentrated solutions were measured ( Fig. 4a ). The ultraviolet-visible spectra include the Au 38 -specific electronic transition at 629 nm ( Fig. 3b ). The CD spectra give perfect mirror images and eleven clear signals are observable between 230 and 900 nm (245 (+), 255 (+), 308 (+), 345 (−), 393 (−), 440 (+), 479 (−) 564 (+), 629 (−) and 747 (+) nm; signs are given for enantiomer 1 , that is, the first enantiomer eluting from the HPLC column. Compared with the ordinary absorption spectrum of Au 38 (SR) 24 , which is highly structured showing several peaks and shoulders, more distinct transitions can be identified in the CD. The identified peaks are in good agreement with those reported for absorption spectra at low temperatures [44] . Anisotropy factors g = ΔA/A = θ [mdeg]/(32980× A) were calculated over the spectral range ( Fig. 4b ). Surprisingly, these are quite strong with values between 1×10 −3 and up to 4×10 −3 ; notably, the anisotropy factor increases with increasing wavelength (decreasing energy). The maximum anisotropy factor of gold nanoclusters protected with chiral thiols was reported to be up to 4×10 −3 (ref. 24 ). This indicates that intrinsic chirality due to ligand arrangement can contribute significantly to the net optical activity. 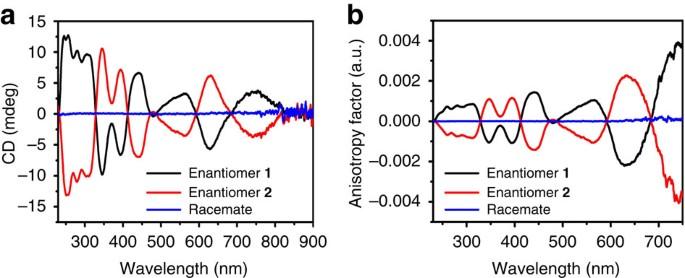Figure 4: CD spectra and anisotropy factors of Au38(SCH2CH2Ph)24. (a) CD spectra of isolated enantiomers1(black) and2(red) and the racemic Au38(SCH2CH2Ph)24(blue) before separation; (b) corresponding anisotropy factors of enantiomers1and2and of the racemate. The spectra exhibit excellent mirror-image relationships and anisotropy factorsg=ΔA/A of up to 4×10−3. Figure 4: CD spectra and anisotropy factors of Au 38 (SCH 2 CH 2 Ph) 24 . ( a ) CD spectra of isolated enantiomers 1 (black) and 2 (red) and the racemic Au 38 (SCH 2 CH 2 Ph) 24 (blue) before separation; ( b ) corresponding anisotropy factors of enantiomers 1 and 2 and of the racemate. The spectra exhibit excellent mirror-image relationships and anisotropy factors g =ΔA/A of up to 4×10 −3 . Full size image Comparison of the chiroptical properties of the intrinsically chiral Au 38 with those reported for Au 38 clusters with chiral thiols is self-evident, as it gives direct insight into the contribution of a chiral ligand to the shape and strength of the CD spectra. Schaaff and Whetten reported a series of glutathionate-protected Au clusters that were separated by gel electrophoresis [18] . The absorption features of compound 3 in ref. 18 are in good agreement with those of Au 38 clusters, although the assignment is not made in the report. Interestingly, the energies and signs of the peak maxima are in very good agreement with those of enantiomer 2 of Au 38 (SCH 2 CH 2 Ph) 2 ( Table 1 ). Minor differences occur for ultraviolet transitions (below 300 nm). In this region, the glutathionate-ligand should contribute to the CD spectrum. Of note, the maximum anisotropy factors of Au 38 (SCH 2 CH 2 Ph) 24 (4×10 −3 ) exceed those of Au 38 (SG) 24 (1.3×10 −3 ), but this could be due to parameters such as solvent or sample purity after gel electrophoresis. However, for most of the spectral range, the anisotropy factors are similar. This indicates that (in this case) the chiral ligand does not have the dominant influence on the chiroptical properties of Au 38 clusters. We doubt that this finding can be generalized as chiral ligands can induce optical activity to clusters that are not intrinsically chiral (such as Au 25 (SR) 18 ) [17] , [27] . The good agreement between the CD spectra of Au 38 (SCH 2 CH 2 Ph) 24 and Au 38 ( L -SG) 24 strongly indicates that, in the latter case, one-handedness of the cluster (which dominated the CD spectra in the Au 38 case) is favoured over the other due to the presence of the chiral glutathionate-ligand. In other words, there is a strong diastereoselectivity during the formation of Au 38 ( L -SG) 24 . Table 1 Wavelengths, anisotropy factors, and signs of enantiomer 2 of Au 38 (SCH 2 CH 2 Ph) 24 , Au 38 (SG) 24 (ref. 18 ) and Au 38 (SMe) 24 (ref. 6 ). Full size table In a recent article, Lopez-Acevedo et al . simulated the structure, and predicted the intrinsic chirality of Au 38 (SR) 24 (ref. 6 ). Moreover, the CD spectra of the cluster were computed for the right-handed enantiomer (structure 1 in ref. 6 was identified as being the 'correct' structure). Comparison of the experimental spectra with those computed (with methylthiolate as model ligand) shows a good match for the spectral range from 800 to 500 nm available for comparison with transitions at 747, 629 and 564 nm (a comparison of a wider range is not possible as it was either not measured (lower energies) or not presented in the figures (higher energies)). Moreover, the experimental and calculated anisotropy factors are of similar magnitudes ( Table 1 ). As the sign of the calculated spectrum agrees with the experimental spectrum of enantiomer 2, we tentatively assign the latter as the right-handed one. Comparison of the spectra of Au 38 (SCH 2 CH 2 Ph) 24 with Au 38 (SG) 24 and (simulated) Au(SMe) 24 reveals a minor influence of the ligand to the shape of the CD spectra as all three spectra are in good agreement concerning energies, sign and magnitude of anisotropy. As it is possible to separate the enantiomers and measure CD spectra of good quality, no racemization is thought to occur over several hours in solution (the sum of the anisotropy factor plots gives a zero line, indicating the same enantiomeric excess in both fractions). The collected solutions of the two chromatographic fractions were concentrated to dryness and stored at −5 °C over 3 days. After that time, the anisotropy factors of the enantiomers were identical to the one measured directly after chromatography, indicating that racemization does not take place under these conditions. In this report, we present the first successful enantioseparation of racemic Au 38 (SR) 24 nanoclusters. Moreover, the studied clusters are protected by achiral ligands (−SCH 2 CH 2 Ph) and the observed chirality is an intrinsic structural property of the cluster. The observed optical activity is the first spectroscopic evidence of chirality stemming only from the asymmetric arrangement of achiral adsorbates on a surface. This type of chirality has been identified by X-ray diffraction and, in the case of extended surfaces, by microscopy studies [1] , [2] , [3] , [4] . The observed anisotropy factors of up to 4×10 −3 are surprisingly strong, considering the fact that no chiral ligands are present. Comparison with glutathionate-protected Au 38 clusters only shows a minor influence of the chiral ligand to the spectrum (indicating that one enantiomer is selectively formed when glutathione is used) [18] . Moreover, the spectrum is in good qualitative and quantitative agreement with those of computed structures [6] . General All chemicals were used as received, if not mentioned otherwise. Tetrachloroauric acid trihydrate (Aldrich, 99.9+%), reduced L -glutathione (Sigma-Aldrich, >99%), sodium borohydride (Fluka, >96%), 2-phenylethylthiol (Aldrich, 98%), anhydrous sodium sulfate (Reactolab, Servion/CH), [3-(4- tert -butylphenyl)-2-methyl-2-propenylidene]malononitrile (Aldrich, >98%), methanol (VWR, >99.8%), acetone (Fluka, >99.5%), methylene chloride (Sigma-Aldrich, >99.9%), tetrahydrofuran (Acros, p.A. ), hexane (Sigma-Aldrich, HPLC grade), isopropanol (Sigma-Aldrich, HPLC grade), regenerated cellulose membranes (0.2 μm, Sartorius), PTFE syringe filters (0.2 μm, Carl Roth) and Bio Beads SX-1 (Bio-Rad) were used as received, if not mentioned otherwise. Tetrahydrofuran was dried over sodium sulfate and stored under nitrogen. Nanopure water (>18 MΩ) was used. Synthesis and isolation of rac-Au 38 (SCH 2 CH 2 Ph) 24 Step 1. Preparation of L -glutathionate-protected clusters. Tetrachloroauric acid trihydrate (1 g, 2.54 mmol) was dissolved in methanol (200 ml); L -glutathione (3.1 g, 10.18 mmol) was dissolved in water (100 ml). The solutions were combined and stirred at room temperature for 30 min. During this, a yellow-brown suspension was formed. A freshly prepared, ice-cooled solution of sodium borohydride (1.1 g, 30 mmol) in water (60 ml) was added all at once. Immediately, the reaction mixture turned dark-brown to black. The solution was stirred at room temperature for 90 min, during which the clusters precipitated. The solvent was decanted and the crude material was washed with methanol several times. Step 2. Thermal etching towards rac -Au 38 (SCH 2 CH 2 Ph) 24 . The L -glutathionate-protected clusters from Step 1 (ca 550 mg) were dissolved in 10 ml of water and 10 ml of acetone and 15 ml of 2-phenylethylthiol were added. The mixture was stirred at 80 °C for 3 h, during which the aqueous phase discoloured. Some insoluble white material formed. The crude reaction mixture was diluted with water and extracted with methylene chloride. The aqueous phase was discarded. The solvent was removed from the organic phase and the clusters were extensively washed with methanol to remove excess thiol and other byproducts and filtered over a regenerated cellulose filter (0.2 μm). Clusters were redissolved in methylene chloride and methanol precipitation and washing was repeated. Overall, five washing cycles were applied. Eventually, the clusters were dissolved in methylene chloride and passed through a PTFE syringe filter (0.2 μm) to remove insoluble byproducts. After this, ultraviolet-visible and MALDI mass spectra were recorded. Step 3—Size-selection of rac -Au 38 (SCH 2 CH 2 Ph) 24 . A weight of 45 g of Bio-Rad BioBeads SX-1 was suspended in about 7 times the bed volume of tetrahydrofuran. The beads were allowed to swell overnight and given into a glass column (100 cm in length and 2.5 cm in diameter) equipped with a glass frit (G4) and inert gas inlet. The beads were allowed to settle (90 cm bed height) under a gentle stream of N 2 and washed extensively with tetrahydrofuran (ca 500 ml). The crude clusters from Step 2 were dissolved in a minimum amount of tetrahydrofuran and repeatedly eluted, using tetrahydrofuran as mobile phase (ca 1 ml min −1 ) until the eluting clusters were purely composed of Au 38 (SCH 2 CH 2 Ph) 24 (the eluting band overlaps with Au 40 (SCH 2 CH 2 Ph) 24 ; therefore, repeated chromatographic separations are necessary.). The collected fractions were characterized by ultraviolet-visible spectroscopy, until no further change was observed. The fraction identified as rac -Au 38 (SCH 2 CH 2 Ph) 24 was washed with methanol and passed over a PTFE syringe filter, as described in Step 2 before characterization with ultraviolet-visible and CD spectroscopy as well as MALDI mass spectrometry. Ultraviolet-visible spectroscopy Ultraviolet-visible spectra were recorded on a Varian Cary 50 spectrophotometer, using a quartz cuvette of 10 and 5 mm path length. Spectra were measured in methylene chloride and normalized at 300 nm. CD spectroscopy CD spectra were recorded on a JASCO J-815 CD-spectrometer using a quartz cuvette of 5 mm path length. The spectra were recorded in diluted solutions of methylene chloride and the signal of the blank solvent was subtracted. For each spectrum, eight scans at a scanning speed of 100 nm/min at a data pitch of 0.1 nm were averaged. The spectra were recorded at 20 °C; for temperature control, a JACSO PFD-350S Peltier element was used. Anisotropy factors g = θ [mdeg]/(32980 × A) were calculated using the ultraviolet-visible spectrum provided by the CD spectrometer. MALDI analysis Mass spectra were obtained using a Bruker Autoflex mass spectrometer equipped with a nitrogen laser at near threshold laser fluence in positive linear mode. [3-(4- tert -Butylphenyl)-2-methyl-2-propenylidene]malononitrile was used as the matrix with a 1:1,000 analyte : matrix ratio [42] . A volume of 2 μl of the analyte/matrix mixture was applied to the target and air-dried. HPLC Chromatographic separation of the enantiomers was achieved on a JASCO 20XX HPLC system equipped with a Phenomenex Lux-Cellulose-1 column (5 μm, 250 mm×4.6 mm). For detection, a JASCO 2070plus ultraviolet-visible detector was used. Path length was 10 mm and the wavelength was set to 380 nm. The analytes were eluted at a flow rate of 2 ml min −1 using hexane:isopropanol (80:20). For separation at different temperatures, a Thermasphere TS-430 HPLC column chiller/heater was used. How to cite this article: Dolamic, I. et al . First enantioseparation and circular dichroism spectra of Au 38 clusters protected by achiral ligands. Nat. Commun. 3:798 doi: 10.1038/ncomms1802 (2012).